Twist1 induces endothelial differentiation of tumour cells through the Jagged1-KLF4 axis The mechanisms controlling tumour-induced angiogenesis are presently not clear. In principle, angiogenesis can be achieved through the activation of endothelial cells in existing vessels or by transdifferentiation of tumour cells into endothelial cells. However, whether tumour cells can go through a prior epithelial–mesenchymal transition and further differentiate into endothelial cells remains unknown. Here we show that overexpression of Twist1, a transcriptional regulator that induces and promotes cancer metastasis, leads to endothelial differentiation in head and neck cancer (HNC) cells. Induction of Jagged1 expression by Twist1 is essential for Twist1-induced endothelial differentiation. The Jagged1/Notch signalling subsequently activates KLF4, inducing stem-like properties in HNC cells and conferring them with drug resistance. Our results indicate that the Twist1-Jagged1/KLF4 axis is essential both for transdifferentiation of tumour cells into endothelial cells and for chemoresistance acquisition. Tumour angiogenesis is one of the hallmark capabilities that enable tumour growth and metastasis [1] . The endothelial cells that constitute tumour vasculature can be generated from the existing endothelial cells through the ‘angiogenic switch’ mediated by different signalling molecules [2] , [3] . Alternatively, endothelial stem-like cells with cancer-specific genomic alterations have been described in different tumour types [4] , [5] . Recently, transdifferentiation of glioblastoma stem-like cells into endothelial cells has been demonstrated [6] , [7] , [8] . However, it is unknown whether tumour cells can go through a prior epithelial–mesenchymal transition (EMT) before further differentiation into endothelial cells. Twist1, a master transcriptional regulator of mesoderm development, induces EMT and promotes cancer metastasis [9] , [10] , [11] , [12] . Twist1 overexpression is observed in many different types of human cancers [12] . The Notch signalling not only regulates vascular morphogenesis but also communicates with existing endothelial cells to promote tumour angiogenesis [13] , [14] , [15] . KLF4 is a core component of the pluripotency transcription network that has been used to reprogram somatic cells into induced pluripotent stem cells [16] . KLF4 regulates endothelial barrier and is implicated in vasculogenesis [17] , [18] . Recent evidence has shown that pluripotency factors regulate endoderm specification [19] . The precise role of KLF4 in the induction of endothelial differentiation remains to be determined. In this report, we explore the ability of Twist1 to induce endothelial differentiation of tumour cells after these cells have gone through EMT. The signalling pathways of tumour-derived endothelial differentiation induced by Twist1 are also investigated, which are involved in the induction of stem-like property and drug resistance. These results provide a fresh insight into the mechanisms of endothelial differentiation and chemoresistance mediated by Twist1 and endow Twist1-overexpressing tumours with a promising implication of treatment. Twist1 induces endothelial differentiation of tumour cells To test the ability of Twist1 to induce endothelial differentiation of tumour cells, we overexpressed Twist1 in a head and neck cancer (HNC) cell line, OECM1, and examined the expressions of endothelial markers, including CD31 and CD144 [6] , [7] , [8] . Western blot analysis showed that CD31 and CD144 were activated in Twist1-overexpressing OECM1 cells and about 10% of Twist1-overexpressing cells expressed CD31 and CD144 as determined by flow cytometry ( Fig. 1a ; Supplementary Fig. 1a ). The increased expression of CD31 and CD144 is independently validated in another HNC cell line, FADU with Twist1 overexpression ( Supplementary Fig. 1b,c ). About 10% of Twist1-overexpressing OECM1 cells co-expressed CD144 ( Fig. 1b ) and ~9% co-expressed vimentin and CD144 ( Supplementary Fig. 2a ). Further sorting by flow cytometry revealed that among Twist1-overexpressing OECM1 cells, those (9–10%) co-expressed with CD144 or CD31 had the highest levels of Twist1 ( Supplementary Fig. 2b,c ). However, induction of CD31 and CD144 by Twist1 overexpression was not mediated through chemokine receptor 4 (CXCR4) since CXCR4 was not activated by Twist1 ( Supplementary Fig. 2d ). Twist1-overexpressing OECM1 cells exhibited increased tube-forming ability, haemoglobin levels in xenografted tumours and DiI-AcLDL (1,1′-dioctadecyl-3,3,3′,3′-tetramethyl-indocarbocyanide perchlorate-labelled acetylated low-density lipoproteins) uptake [8] ( Fig. 1c,d ; Supplementary Fig. 2e ). Other endothelial markers, including von Willebrand factor (vWF), TEK tyrosine kinase (TIE2), CD105 and intercellular adhesion molecule 1 (ICAM1), [6] , [7] , [20] were also activated by Twist1 overexpression and western blot analysis confirmed the activation of CD105 and ICAM1 in Twist1-overexpressing OECM1 cells ( Fig. 2a–c ). Examination of different vascular markers by real-time PCR analysis showed the increased expression of ephrin B2 ( EFNB2) and neuropilin 1 ( NRP1) and decreased expression of EPH receptor B4 (EPHB4) in Twist1-overexpressing OECM1 cells ( Fig. 2d ). The Twist1-overexpressing and the control OECM1 cells were labelled with green fluorescence protein (GFP) followed by subcutaneous injection into nude mice to monitor tumour vessel formation in xenografted tumours. The results showed that Twist1-overexpressing OECM1 cells contributed to the formation of tumour vessels as determined by the co-staining of CD144 and GFP ( Fig. 1e ). The GFP and CD144 co-expressing tumour vessels were located mostly inside the tumour mass. The hemotoxylin and eosin (H&E) staining of consecutive slides also showed the vascular structure ( Supplementary Fig. 3a ). Finally, immunofluorescence staining of Twist1 and CD31 showed that 91.6% (22/24) of Twist1-overexpressing HNC patient samples had tumour-derived vessel formation as determined by the co-expression of CD31 and Twist1 in the same cells ( Fig. 1f ). Immunofluorescence staining of CD144 and Twist1 also showed the co-staining of both markers in patient samples ( Supplementary Fig. 3c ). The H&E staining of consecutive slides showed the vascular structure ( Supplementary Fig. 3b,c ). Consistent with the above results, knockdown of Twist1 in H1299 (non-small cell lung cancer) and SAS (HNC) cells decreased the tube-forming ability and CD31 levels, and inhibited DiI-AcLDL uptake ( Supplementary Figs 4 and 5a,b ). Moreover, haemoglobin (Hb) levels were decreased in xenografted tumours when Twist1 was knocked down in H1299 cells ( Supplementary Fig. 5c ), suggesting that endothelial differentiation was reduced in vivo . In support of this finding, expression of the endothelial markers (CD31, vWF, TIE2 and CD105) was repressed in Twist1-knockdown H1299 and SAS cells (left panels in Supplementary Fig. 6a,b ). Noticeably, the expression pattern of vascular markers (EFNB2, NRP1, EPHB4) was also consistent with the Twist1 overexpression status (right panels in Supplementary Fig. 6a,b ). Finally, due to the causative role of human papilloma virus (HPV) in HNC formation [21] , we tested whether there was a correlation between HPV infection and Twist1 overexpression. The result showed that there was no significant correlation between the presence of HPV and Twist1 overexpression in patient samples ( Supplementary Fig. 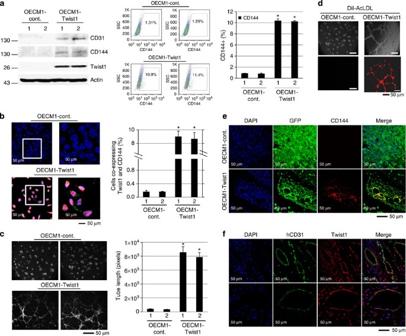Figure 1: Induction of tumour-derived endothelial differentiation by Twist1. (a) Expression of CD31 and CD144 in Twist1-overexpressing OECM1 cells using western blot analysis. The middle panel showed the dot plots from flow cytometry analysis and the rightmost panel showed the percentage of cells expressing CD144 in Twist1-overexpressing OECM1 cells. (b) Co-expression of Twist1 and CD144 in Twist1-overexpressing OECM1 cells. Red: Twist1; green: CD144. (Left panels: images; right panel: the percentage of cells co-expressing Twist1 and CD144.) Scale bar, 50 μm. (c) 2.5-Dimensional (2.5D) tube-forming ability assays in Twist1-overexpressing OECM1 cells (left panels: images; right panel: pixels representing tube formation as described in Methods section (bar graph)). Scale bar, 50 μm. (d) DiI-AcLDL uptake assays in Twist1-overexpressing OECM1 cells. Red: DiI-AcLDL staining. The AcLDL staining photos were accompanied by 3D tube-formation ability photos (on top of Dil-AcLDL staining) for each clone. Scale bar, 50 μm. (e) Participation of GFP-labelled Twist1-overexpressing cells in tumour vessel formation. Green: GFP; red: CD144; blue: DAPI. Scale bar, 50 μm. (f) Co-expression of Twist1 and CD31 in HNC patient samples. Examples from two different patient samples are shown. Green: hCD31; red: Twist1; blue: DAPI. Scale bar, 50 μm. Data shown in panelsa–care mean±s.d. of three independent experiments. Asterisk (*) indicates statistical significance (P<0.05 by Student’st-test) between experimental and control (cont.) clones. The OECM1 control clone was selected as the control group in panelsa–c. 5d ; Supplementary Table 1 ). These results indicate that Twist1 overexpression induces endothelial differentiation of tumour cells that favours arterial specification [22] , [23] and promotes tumour vascular formation. Figure 1: Induction of tumour-derived endothelial differentiation by Twist1. ( a ) Expression of CD31 and CD144 in Twist1-overexpressing OECM1 cells using western blot analysis. The middle panel showed the dot plots from flow cytometry analysis and the rightmost panel showed the percentage of cells expressing CD144 in Twist1-overexpressing OECM1 cells. ( b ) Co-expression of Twist1 and CD144 in Twist1-overexpressing OECM1 cells. Red: Twist1; green: CD144. (Left panels: images; right panel: the percentage of cells co-expressing Twist1 and CD144.) Scale bar, 50 μm. ( c ) 2.5-Dimensional (2.5D) tube-forming ability assays in Twist1-overexpressing OECM1 cells (left panels: images; right panel: pixels representing tube formation as described in Methods section (bar graph)). Scale bar, 50 μm. ( d ) DiI-AcLDL uptake assays in Twist1-overexpressing OECM1 cells. Red: DiI-AcLDL staining. The AcLDL staining photos were accompanied by 3D tube-formation ability photos (on top of Dil-AcLDL staining) for each clone. Scale bar, 50 μm. ( e ) Participation of GFP-labelled Twist1-overexpressing cells in tumour vessel formation. Green: GFP; red: CD144; blue: DAPI. Scale bar, 50 μm. ( f ) Co-expression of Twist1 and CD31 in HNC patient samples. Examples from two different patient samples are shown. Green: hCD31; red: Twist1; blue: DAPI. Scale bar, 50 μm. Data shown in panels a – c are mean±s.d. of three independent experiments. Asterisk (*) indicates statistical significance ( P <0.05 by Student’s t -test) between experimental and control (cont.) clones. The OECM1 control clone was selected as the control group in panels a – c . 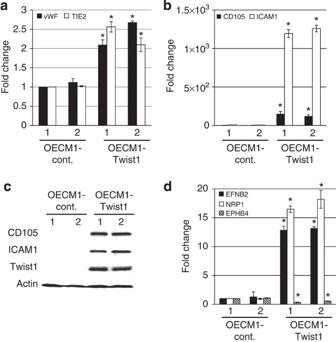Figure 2: Regulation of various endothelial and vascular markers by Twist1. (a,b) Real-time PCR analysis of various endothelial markers including vWF, TIE2, CD105 and ICAM1 in Twist1-overexpressing OECM1 clones. Fold change of relative RNA expression was shown (bar graph). (c) Western blot analysis of CD105 and ICAM1 in Twist1-overexpressing OECM1 cell clones versus the control (cont.) clones. (d) Real-time PCR analysis of various vascular markers including EFNB2, NRP1 and EPHB4 in Twist1-overexpressing OECM1 clones. The OECM1 control clone was selected as the control group in panelsa–d. Data shown in panelsa,b,dare mean±s.d. of three independent experiments. Asterisk (*) indicates statistical significance (P<0.05 by Student’st-test) between experimental and control clones. Full size image Figure 2: Regulation of various endothelial and vascular markers by Twist1. ( a , b ) Real-time PCR analysis of various endothelial markers including vWF, TIE2, CD105 and ICAM1 in Twist1-overexpressing OECM1 clones. Fold change of relative RNA expression was shown (bar graph). ( c ) Western blot analysis of CD105 and ICAM1 in Twist1-overexpressing OECM1 cell clones versus the control (cont.) clones. ( d ) Real-time PCR analysis of various vascular markers including EFNB2, NRP1 and EPHB4 in Twist1-overexpressing OECM1 clones. The OECM1 control clone was selected as the control group in panels a – d . Data shown in panels a , b , d are mean±s.d. of three independent experiments. Asterisk (*) indicates statistical significance ( P <0.05 by Student’s t -test) between experimental and control clones. Full size image Twist1 induced Jagged1 to mediate endothelial differentiation To explore the mechanism that mediates induction of endothelial differentiation by Twist1, a microarray approach was performed to search for putative Twist1 downstream targets. Among the putative Twist1 targets, we chose a Notch ligand, Jagged1, since Notch signalling regulates tumour angiogenesis [13] , [14] . Further confirmation using real-time PCR and western blot showed that Twist1 overexpression induced the expressions of Jagged1 and its downstream targets, Hes1 , Hey1 and Hey 2 ( Supplementary Fig. 7a,b ) [13] . Knockdown of Twist1 in H1299 cells reduced the expression of Jagged1, Hes1, Hey1 and Hey2 ( Supplementary Fig. 7c,d ), suggesting that the same signalling pathway existed in a different cell type. To test a direct activation of Jagged1 by Twist1, we identified a Twist1-binding site in the Jagged1 promoter using transient transfection assays ( Fig. 3a,b ). Chromatin immunoprecipitation (ChIP) experiments showed the direct binding of Twist1 to the Jagged1 promoter in two different cell lines ( Fig. 3c ). To test the role of Jagged1 in Twist1-induced endothelial differentiation, we knocked down Jagged1 in Twist1-overexpressing OECM1 cells and this led to a decrease in CD31 and CD144 expressions and DiI-AcLDL uptake ( Fig. 4a ; Supplementary Fig. 8 ). Knockdown of Jagged1 also decreased haemoglobin (Hb) levels in xenografted tumours, the tube-formation ability and the expression of CD31, CD144, vWF, CD105 and ICAM1 induced by Twist1 overexpression ( Fig. 4b,c ; Supplementary Fig. 9 ). In addition, we examined various vascular markers in these cells and found that Jagged1 knockdown reduced the mRNA levels of EFNB2 , NRP1 and EPHB4 ( Fig. 4d ), indicating the essential role of Jagged1 in Twist1-mediated regulation of vascular markers. Knockdown of Jagged1 also decreased the percentage of GFP- and CD144-co-staining cells or CD31- and Twist1-co-expressing cells ( Fig. 4e,f ). The H&E staining of consecutive sections was shown ( Supplementary Fig. 10 ). Finally, to test whether Jagged1 is involved in Twist1-induced metastasis, in vitro migration/invasion assays were performed. The results showed that Jagged1 knockdown in Twist1-overexpressing OECM1 or H1299 cells reversed EMT and decreased the in vitro metastatic activity induced by Twist1 ( Supplementary Fig. 11 ). Together, these results indicate an essential role of Jagged1 in Twist1-induced endothelial differentiation, EMT and metastasis. 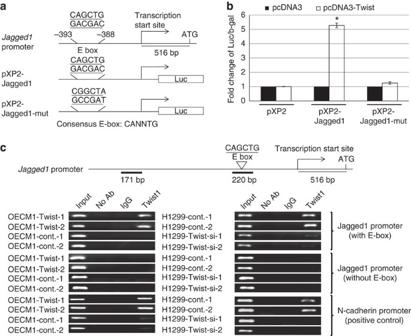Figure 3: Direct activation ofJagged1expression by Twist1. (a) The promoter region of theJagged1gene containing a putative Twist1-responsive site. (b) Transient transfection experiments were performed using a Twist1 expression vector with aJagged1promoter-driven reporter construct harbouring either a wild-type or mutated Twist1-responsive site. The pcDNA3 control-transfected lane was selected as the control group versus the pcDNA3-Twist1-transfected lane for each reporter construct. Data shown in panelbare mean±s.d. of three independent experiments. Asterisk (*) indicates statistical significance (P<0.05 by Student’st-test) between experimental and control clones. (c) ChIP experiments were performed using the IgG or anti-Twist1 antibody to detect their binding to two regions in theJagged1gene promoter. Two different cell lines (OECM1, H1299) with different Twist1 expression status were tested. The binding of Twist1 to theN-cadherinpromoter was used as a positive control. Figure 3: Direct activation of Jagged1 expression by Twist1. ( a ) The promoter region of the Jagged1 gene containing a putative Twist1-responsive site. ( b ) Transient transfection experiments were performed using a Twist1 expression vector with a Jagged1 promoter-driven reporter construct harbouring either a wild-type or mutated Twist1-responsive site. The pcDNA3 control-transfected lane was selected as the control group versus the pcDNA3-Twist1-transfected lane for each reporter construct. Data shown in panel b are mean±s.d. of three independent experiments. Asterisk (*) indicates statistical significance ( P <0.05 by Student’s t -test) between experimental and control clones. ( c ) ChIP experiments were performed using the IgG or anti-Twist1 antibody to detect their binding to two regions in the Jagged1 gene promoter. Two different cell lines (OECM1, H1299) with different Twist1 expression status were tested. The binding of Twist1 to the N-cadherin promoter was used as a positive control. 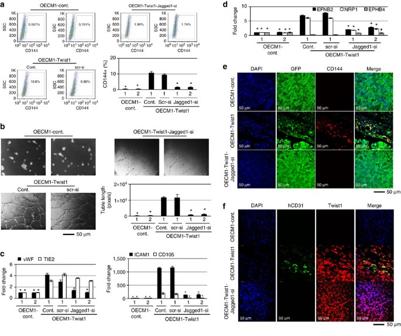Figure 4: Jagged1 is essential for Twist1-induced endothelial differentiation. (a) Expression of CD144 in Twist1-overexpressing OECM1 cells with knockdown of Jagged1. Dot plots from flow cytometry and the percentage of cells expressing CD144 (bar graph) are shown. (b) 2.5-Dimensional (2.5D) tube-formation ability assays in Twist1-overexpressing OECM1 cells with knockdown of Jagged1. Images of tube formation and pixels representing tube-formation ability (bar graph) are shown. Scale bar, 50 μm. (c) Expression of various endothelial markers including vWF, TIE2, ICAM1 and CD105 in Twist1-overexpressing OECM1 cells. Fold change of the levels of various endothelial markers was shown. (d) Expression ofEFNB2, NRP1andEPHB4in Twist1-overexpressing OECM1 cells with knockdown of Jagged1. (e) Expression of CD144 in GFP-labelled Twist1-overexpressing OECM1 cells with knockdown of Jagged1. Green: GFP; red: CD144; blue: DAPI. Scale bar, 50 μm. (f) Co-expression of Twist1 and CD31 in Twist1-overexpressing cells with knockdown of Jagged1. Green: hCD31; red: Twist1; blue: DAPI. Data shown in panelsa–dare mean±s.d. of three independent experiments. Asterisk (*) indicates statistical significance (P<0.05 by Student’st-test) between experimental and control (cont.) clones. The OECM1-Twist1 control clone was selected as the control group in panelsa–f. Full size image Figure 4: Jagged1 is essential for Twist1-induced endothelial differentiation. ( a ) Expression of CD144 in Twist1-overexpressing OECM1 cells with knockdown of Jagged1. Dot plots from flow cytometry and the percentage of cells expressing CD144 (bar graph) are shown. ( b ) 2.5-Dimensional (2.5D) tube-formation ability assays in Twist1-overexpressing OECM1 cells with knockdown of Jagged1. Images of tube formation and pixels representing tube-formation ability (bar graph) are shown. Scale bar, 50 μm. ( c ) Expression of various endothelial markers including vWF, TIE2, ICAM1 and CD105 in Twist1-overexpressing OECM1 cells. Fold change of the levels of various endothelial markers was shown. ( d ) Expression of EFNB2, NRP1 and EPHB4 in Twist1-overexpressing OECM1 cells with knockdown of Jagged1. ( e ) Expression of CD144 in GFP-labelled Twist1-overexpressing OECM1 cells with knockdown of Jagged1. Green: GFP; red: CD144; blue: DAPI. Scale bar, 50 μm. ( f ) Co-expression of Twist1 and CD31 in Twist1-overexpressing cells with knockdown of Jagged1. Green: hCD31; red: Twist1; blue: DAPI. Data shown in panels a – d are mean±s.d. of three independent experiments. Asterisk (*) indicates statistical significance ( P <0.05 by Student’s t -test) between experimental and control (cont.) clones. The OECM1-Twist1 control clone was selected as the control group in panels a – f . Full size image Regulation of KLF4 by the Twist1-Jagged1/Notch signalling Transdifferentiation into endothelial cells from tumour stem-like cells [6] , [7] , [8] may be regulated by stemness-related transcription factors. Pluripotency factors have been shown to regulate endoderm specification [19] . To further identify the transcription factors controlled by the Twist1-Jagged1/Notch axis that regulate the expression of various endothelial and vascular marker genes, different stemness-related transcriptional regulators, including OCT4, SOX2, NANOG, KLF4, GFI1, WNT and BMI1, were screened to correlate their expression with the Twist1-Jagged1/Notch axis [16] , [24] . Only KLF4 correlated with the expression of Twist1 and Jagged1 ( Supplementary Fig. 12a ). Real-time PCR and western blot analysis showed that further knockdown of Jagged1 decreased the levels of KLF4 in Twist1-overexpressing OECM1 cells ( Fig. 5a ; Supplementary Fig. 12b ). This correlation was corroborated by another cell line, H1299, in which a decrease in Jagged1 also downregulated KLF4 ( Supplementary Fig. 12c ). To test a direct activation of KLF4 by Jagged1, we transiently transfected Jagged1 with a KLF4 promoter-driven reporter construct harbouring either a wild-type or mutated Notch intracellular domain (NICD)/CSL (CBF1, Suppressor of Hairless, Lag-1)-responsive site. The KLF4 reporter was activated by Jagged1 overexpression, but mutated KLF4 reporter was unresponsive ( Fig. 5b ). Moreover, ChIP experiments showed a direct binding of NICD/CSL to the KLF4 promoter in two different cell lines, whereas Jagged1 depletion abolished this interaction ( Fig. 5c ). Together, these results indicate that KLF4 is a direct target of Jagged1 and its activation is controlled by the Jagged1/Notch signalling. 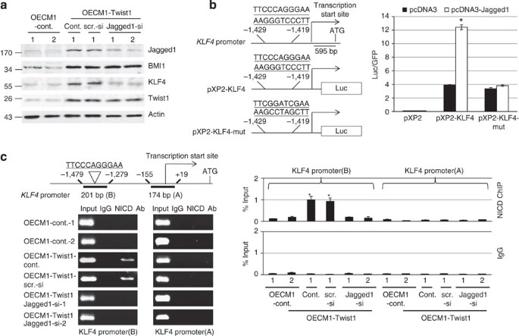Figure 5: Direct activation ofKLF4expression by the Jagged1/Notch signalling. (a) Western blot to examine the expression levels of Jagged1, BMI1, KLF4 and Twist1 in various stable clones. Actin was used as an internal control. (b) Transient transfection assays were performed using a Jagged1 expression vector with aKLF4promoter-driven reporter construct harbouring either a wild-type or mutated NICD/CSL-responsive site. The pcDNA3 control-transfected lane was selected as the control group versus the pcDNA3-Jagged1-transfected lane for each reporter construct. (c) ChIP experiments were performed using an IgG or anti-NICD antibody to detect their binding to two regions in theKLF4gene promoter. The cell clones of OECM1 control (cont.), OECM1-Twist1 and OECM1-Twist1 with Jagged1 knockdown were used. qChIP results of NICD binding to theKLF4promoter regions were also shown. The OECM1 control clone was selected as a control. TheHes1promoter was used as a positive control for NICD binding (Supplementary Fig. 28c). Data shown in panelsb,care mean±s.d. of three independent experiments. Asterisk (*) indicates statistical significance (P<0.05 by Student’st-test) between experimental and control transfections (b) or control clones (c). Figure 5: Direct activation of KLF4 expression by the Jagged1/Notch signalling. ( a ) Western blot to examine the expression levels of Jagged1, BMI1, KLF4 and Twist1 in various stable clones. Actin was used as an internal control. ( b ) Transient transfection assays were performed using a Jagged1 expression vector with a KLF4 promoter-driven reporter construct harbouring either a wild-type or mutated NICD/CSL-responsive site. The pcDNA3 control-transfected lane was selected as the control group versus the pcDNA3-Jagged1-transfected lane for each reporter construct. ( c ) ChIP experiments were performed using an IgG or anti-NICD antibody to detect their binding to two regions in the KLF4 gene promoter. The cell clones of OECM1 control (cont. ), OECM1-Twist1 and OECM1-Twist1 with Jagged1 knockdown were used. qChIP results of NICD binding to the KLF4 promoter regions were also shown. The OECM1 control clone was selected as a control. The Hes1 promoter was used as a positive control for NICD binding ( Supplementary Fig. 28c ). Data shown in panels b , c are mean±s.d. of three independent experiments. Asterisk (*) indicates statistical significance ( P <0.05 by Student’s t -test) between experimental and control transfections ( b ) or control clones ( c ). Full size image KLF4 mediates Twist1-induced endothelial differentiation In addition to the induction of tumour-derived endothelial differentiation by Twist1, our previous results showed that Twist1 activates BMI1 expression to confer stem cell-like property [24] . Since both BMI1 and KLF4 are factors capable of promoting stemness [16] , [24] , we wanted to assign their contribution to Twist1-induced endothelial differentiation. KFL4-, BMI1- or KFL4/BMI1-knockdown clones were generated in Twist1-overexpressing stable cells ( Fig. 6a ). KLF4 or BMI1 knockdown decreased the percentage of CD31+ and CD144+ population in Twist1-overexpressing OECM1 cells by flow cytometry and immunofluorescence staining ( Fig. 6a,b ; Supplementary Fig. 13 ). Increased in vitro tube-formation ability induced by Twist1 was also abolished by either KLF4 or BMI1 knockdown ( Supplementary Fig. 14 ). Other endothelial phenotypes, such as DiI-AcLDL uptake and Hb levels in xenotransplanted tumours, were also abrogated in Twist1-overexpressing cells with KLF4 or BMI1 knockdown ( Fig. 6b ; Supplementary Fig. 15b ). In vivo xenograft assays showed the abrogation of co-expression of Twist1 and CD31 in Twist1-overexpressing cells with KLF4 or BMI1 knockdown ( Supplementary Fig. 15a , including immunofluorescence and H&E staining of consecutive slides). However, expressions of various endothelial markers, including vWF , ICAM1 and CD105, were abolished in KLF4 knockdown but not in BMI1 knockdown Twist1-overexpressing cells using real-time PCR analysis ( Supplementary Fig. 16a ). KLF4, but not BMI1, was also responsible for the regulation of EFNB2 , NRP1 and EPHB4 expressions ( Supplementary Fig. 16b ). To further examine the role of KLF4 in the regulation of various endothelial and vascular markers, quantitative ChIP (qChIP) assays using an anti-KLF4 antibody to screen the promoter regions of various genes with KLF4 binding were performed. The results showed that KLF4 bound to the proximal promoters of CD31 , CD144 , vWF , CD105 , ICAM1 , EFNB2 and EPHB4 genes ( Fig. 6c ; Supplementary Figs 17–20 ), which were mostly consistent with the results from KLF4-knockdown experiments ( Fig. 6a ; Supplementary Figs 13–16 ). Overexpression of KLF4 in OCEM-1 cells activated the expression of CD31, CD144, ICAM1, CD105 and vWF at both the mRNA and the protein levels ( Supplementary Fig. 21a,b ). qChIP experiments showed that BMI1 only bound to the promoters of CD31 and CD144 genes ( Supplementary Figs 21c and 22 ). In addition, the promoter regions of CD31 and CD144 genes bound by BMI1 were different from the regions bound by KLF4 ( Supplementary Figs 21c and 22 ). These results indicate that BMI1 functions through different mechanisms to mitigate the endothelial phenotype (that is, expression of CD31 and CD144, increased DiI-AcLDL uptake and Hb levels), but it does not exert any effect on the expressions of various endothelial or vascular markers regulated by KLF4. The finding that Twist1-Jagged1-KLF4 can induce endothelial differentiation is consistent with our observation that OECM1 cells expressing CD31 and CD144 actually had the highest Twist1 expression levels ( Supplementary Fig. 2b,c ). Next, we tested the correlation among Twist1, Jagged1 and KLF4 in clinical specimens. Immunohistochemistry (IHC) staining of 242 cases of head and neck squamous cell carcinoma (HNSCC) patient samples showed that there was significant correlation between Twist1 and Jagged1/KLF4 expressions as well as between Jagged1 and KLF4 expressions, indicating that the Twist1-Jagged1-KLF4 axis may be present in clinical patient samples ( Supplementary Tables 2 and 3 ; Supplementary Fig. 23a ). Increased expression of the Twist1-Jagged1-KLF4 signalling axis was also confirmed in two out of six primary HNC samples ( Supplementary Fig. 23b ). Finally, we tested whether other KLF family members, including KLF2 and KLF5, may contribute to Twist1-Jagged1-induced endothelial differentiation [17] . However, quantitative real-time PCR analysis showed that knockdown of Jagged1 in Twist1-overexpressing OECM1 cells did not decrease the KLF2 or KLF5 mRNA levels ( Supplementary Fig. 23c ), indicating that KLF2 or KLF5 does not play a role in Twist1-induced endothelial differentiation. 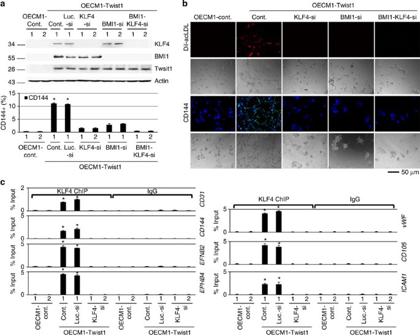Figure 6: KLF4 is essential for Twist1-induced endothelial differentiation. (a) Western blot analysis of KLF4 or BMI1 knockdown or double knockdown clones in Twist1-overexpressing OECM1 cells (upper panel) in OCEM-1 cells overexpressing Twist1. The OECM1-Twist1 control (cont.) clone was selected as the control group. (b) Staining of DiI-AcLDL uptake and CD144 in various clones. The photos of DiL-AcLDL or CD144 staining were accompanied by 3D tube-formation ability photos underneath for each clone. Red: DiI-AcLDL; green: CD144. Scale bar, 50 μm. (c) Binding of KLF4 to the promoters ofCD31, CD144, vWF, CD105, ICAM1, EFNB2andEPHB4genes by qChIP analysis. The promoter regions upstream relative to the transcription start site of each gene that bound KLF4 are:CD31(−1,218 to −1,036 bp);CD144(−218 to −35 bp);EFNB2(+258 to +387 bp);EPHB4(−2,176 to −2,011 bp);vWF(−1,795 to −1,552 bp);CD105(−2,357 to −2,242 bp);ICAM1(−1,187 to −938 bp). The OECM1 control clone was selected as the control group. Data shown in panelsaandcare mean±s.d. of three independent experiments. Asterisk (*) indicates statistical significance (P<0.05 by Student’st-test) between experimental and control clones. Figure 6: KLF4 is essential for Twist1-induced endothelial differentiation. ( a ) Western blot analysis of KLF4 or BMI1 knockdown or double knockdown clones in Twist1-overexpressing OECM1 cells (upper panel) in OCEM-1 cells overexpressing Twist1. The OECM1-Twist1 control (cont.) clone was selected as the control group. ( b ) Staining of DiI-AcLDL uptake and CD144 in various clones. The photos of DiL-AcLDL or CD144 staining were accompanied by 3D tube-formation ability photos underneath for each clone. Red: DiI-AcLDL; green: CD144. Scale bar, 50 μm. ( c ) Binding of KLF4 to the promoters of CD31, CD144, vWF, CD105, ICAM1, EFNB2 and EPHB4 genes by qChIP analysis. The promoter regions upstream relative to the transcription start site of each gene that bound KLF4 are: CD31 (−1,218 to −1,036 bp); CD144 (−218 to −35 bp); EFNB2 (+258 to +387 bp); EPHB4 (−2,176 to −2,011 bp); vWF (−1,795 to −1,552 bp); CD105 (−2,357 to −2,242 bp); ICAM1 (−1,187 to −938 bp). The OECM1 control clone was selected as the control group. Data shown in panels a and c are mean±s.d. of three independent experiments. Asterisk (*) indicates statistical significance ( P <0.05 by Student’s t -test) between experimental and control clones. Full size image KLF4 mediates Twist1-induced stem-like property/metastasis Jagged1 can induce cancer stem cell property with an unknown mechanism [25] . Therefore, we evaluated whether KLF4 and BMI1 contribute to Twist1-induced stem cell-like property due to its tumour-derived endothelial differentiation [6] , [7] , [8] . The analysis of stem cell-like property contained CD44 staining, tumour sphere formation and in vivo tumour-initiating ability assays [24] . The result showed that KLF4 knockdown did not decrease the percentage of CD44+ population induced by Twist1, whereas knockdown of BMI1 abolished the CD44+ population induced by Twist1 (ref. 24 ) ( Supplementary Fig. 24a ). However, knockdown of either KLF4 or BMI1 significantly decreased the size and/or numbers of tumour sphere formation as well as in vivo tumour-initiating ability ( Fig. 7a,b ; Table 1 ; Supplementary Fig. 24b ), suggesting that both BMI1 and KLF4 may contribute to tumour-initiating ability induced by Twist1. Specifically, real-time PCR analysis showed that KLF4 was responsible for the expression of stemness genes ( Wnt5A and CCND2 ) that may control the tumour-initiating ability regulated by KLF4 ( Fig. 7c,d ) [26] , [27] , [28] . The qChIP assay also showed the binding of KLF4 to the promoter regions of Wnt5A gene ( Supplementary Fig. 25a ). These findings suggest that both KLF4 and BMI1 may promote stemness-like property induced by Twist1, but they may regulate cell stemness in a differential way, which needs to be further characterized. 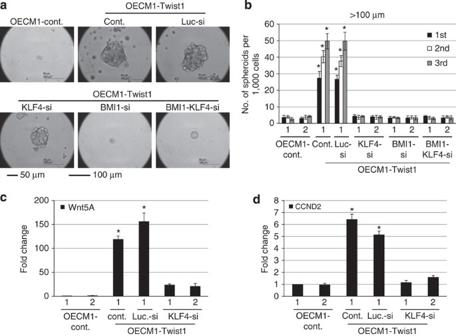Figure 7: Knockdown of KLF4 decreased stem-like property induced by Twist1. (a) Representative pictures of tumour sphere formation of various clones. Scale bar, 50 and 100 μm. (b) Analysis of tumour sphere-formation activity of various clones measured by primary, secondary and tertiary spheres. The number of tumour spheres formed after plating 1,000 cells was measured (bar graph). (c,d) The mRNA expression levels of two stemness genes,Wnt5A(c) andCCND2(d), were measured in various clones using real-time PCR analysis (bar graph). Data shown in panelsb–dare mean±s.d. of three independent experiments. Asterisk (*) indicates statistical significance (P<0.05 by Student’st-test) between experimental and OECM1 control (cont.) clones. Figure 7: Knockdown of KLF4 decreased stem-like property induced by Twist1. ( a ) Representative pictures of tumour sphere formation of various clones. Scale bar, 50 and 100 μm. ( b ) Analysis of tumour sphere-formation activity of various clones measured by primary, secondary and tertiary spheres. The number of tumour spheres formed after plating 1,000 cells was measured (bar graph). ( c , d ) The mRNA expression levels of two stemness genes, Wnt5A ( c ) and CCND2 ( d ), were measured in various clones using real-time PCR analysis (bar graph). Data shown in panels b – d are mean±s.d. of three independent experiments. Asterisk (*) indicates statistical significance ( P <0.05 by Student’s t -test) between experimental and OECM1 control (cont.) clones. Full size image Table 1 In vivo tumour-initiating ability of various clones. Full size table To examine the role of KLF4 in the regulation of EMT marker gene expression [29] , western blot analysis of various clones showed that knockdown of KLF4 did not reverse the EMT marker gene changes induced by Twist1, but knockdown of BMI1 did ( Supplementary Fig. 25b ). However, knockdown of KLF4 still decreased the in vitro migration and invasion activity induced by Twist1 ( Supplementary Fig. 25c ), indicating that KLF4 regulates metastatic activity independent of the EMT marker gene changes. In vivo metastasis assays also showed consistent results with the in vitro migration and invasion assays ( Fig. 8 ). 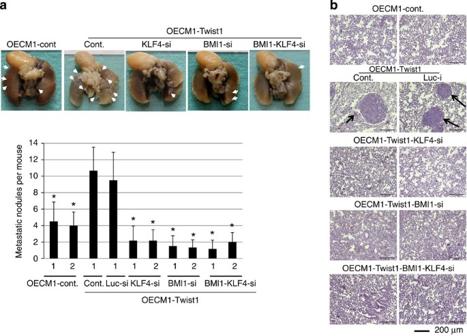Figure 8: The role of KLF4 and BMI1 in Twist1-inducedin vivometastatic activity. (a,b) Gross and histology pictures of lung metastatic nodules generated by injecting various stable clones. (c) Measurement of the number of metastatic lung tumour nodules (bar graph). The OECM1-Twist1 clone was selected as the control group. Luc-si: siRNA against the luciferase gene as a negative control. Data shown in panelcare mean±s.d. of five mice injected with various stable clones in each group. Asterisk (*) indicates statistical significance (P<0.05 by Student’st-test) between experimental and OECM1-Twist1 control (cont.) clones. Figure 8: The role of KLF4 and BMI1 in Twist1-induced in vivo metastatic activity. ( a , b ) Gross and histology pictures of lung metastatic nodules generated by injecting various stable clones. ( c ) Measurement of the number of metastatic lung tumour nodules (bar graph). The OECM1-Twist1 clone was selected as the control group. Luc-si: siRNA against the luciferase gene as a negative control. Data shown in panel c are mean±s.d. of five mice injected with various stable clones in each group. Asterisk (*) indicates statistical significance ( P <0.05 by Student’s t -test) between experimental and OECM1-Twist1 control (cont.) clones. Full size image A strategy for the treatment of Twist1-overexpressing tumours To determine whether the information of Twist1-Jagged1-KLF4 axis can provide a guide to specific treatment strategy for patients with Twist1-overexpressing cancers, Twist1-overexpressing OECM1 cells were used to test drug response. Two commonly used drugs for HNC treatment, cetuximab and cisplatin [30] , [31] , were individually tested with or without a γ-secretase inhibitor N -[ N -(3,5-Difluorophenacetyl)-L-alanyl]-S-phenylglycine t-butyl ester (DAPT) that inhibits Notch signalling [32] . Overexpression of Twist1 increased the viability of cells treated with either cetuximab or cisplatin that could be abolished by KLF4 knockdown ( Supplementary Fig. 26a,b ). Treatment with DAPT together with either cetuximab or cisplatin additively inhibited the viability of Twist1-overexpressing OECM1 cells as well as modulated the expression of endothelial and vascular markers regulated by Twist1 ( Fig. 9a ; Supplementary Figs 26c and 27 ). KLF4 knockdown or DAPT treatment significantly decreased the KLF4+/CD44+ population in Twist1-overexpressing OECM1 cells ( Fig. 9b ). In contrast, treatment with cetuximab or cisplatin did not significantly change the percentage of cells stained with BMI1 or KLF4 ( Fig. 9b ; Supplementary Fig. 26d ). Treatment of xenotransplanted head and neck tumours with cetuximab and DAPT also had an additive tumour-inhibiting effect ( Fig. 9c ; Supplementary Fig. 28a ). These results point to the advantage of using γ-secretase inhibitors (for example, DAPT) in combination with chemotherapy to treat Twist1-overexpressing human tumours. 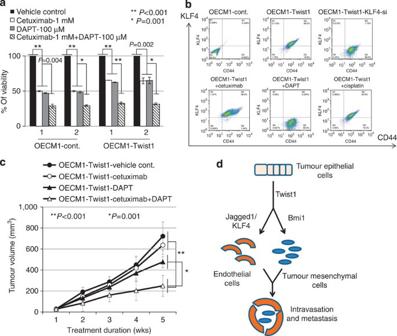Figure 9: Additive tumour-killing effects of DAPT with cetuximab through abolishing the KLF4+ population and a model to summarize the discovery in this report. (a) Tumour-killing effects of DAPT and cetuximab using cell viability assays (the percentage of live cells after drug treatment; bar graph). Data shown are mean±s.d. of three independent experiments. Statistical significance (Student’st-test) was indicated as * or ** between different groups. (b) Flow cytometry analysis of cell population staining with KLF4 and CD44 under different combinations of drug treatment. (c) Xenotransplantation experiments were performed to measure the tumour volume of mice injected with various drugs to determine the tumour-inhibiting effects of various drug treatment (single or combined). Data shown in panelcis mean±s.d. of five mice for each group. Statistical significance (Student’st-test) was indicated as * or ** between different groups. (d) A model to depict the crucial role of the Jagged1-KLF4 axis to mediate endothelial differentiation and form tumour vasculature to support the metastatic process initiated by the induction of EMT by Twist1. cont, control. Figure 9: Additive tumour-killing effects of DAPT with cetuximab through abolishing the KLF4+ population and a model to summarize the discovery in this report. ( a ) Tumour-killing effects of DAPT and cetuximab using cell viability assays (the percentage of live cells after drug treatment; bar graph). Data shown are mean±s.d. of three independent experiments. Statistical significance (Student’s t -test) was indicated as * or ** between different groups. ( b ) Flow cytometry analysis of cell population staining with KLF4 and CD44 under different combinations of drug treatment. ( c ) Xenotransplantation experiments were performed to measure the tumour volume of mice injected with various drugs to determine the tumour-inhibiting effects of various drug treatment (single or combined). Data shown in panel c is mean±s.d. of five mice for each group. Statistical significance (Student’s t -test) was indicated as * or ** between different groups. ( d ) A model to depict the crucial role of the Jagged1-KLF4 axis to mediate endothelial differentiation and form tumour vasculature to support the metastatic process initiated by the induction of EMT by Twist1. cont, control. Full size image Although Twist1 is a master regulator of mesoderm development [9] , our results showed that Twist1 can also induce tumour-derived endothelial differentiation and promote tumour vascular formation. Therefore, the phenomenon of EMT induced by Twist1 [11] , [12] can be extended to the epithelial–mesenchymal–endothelial transition due to co-staining of vimentin (a mesenchymal marker) and CD144 (an endothelial marker) in the same Twist1-overexpressing head and neck tumour cells ( Supplementary Fig. 2a ), suggesting that ~10% of Twist1-overexpressing tumour cells can be driven into endothelial differentiation and contribute directly to the angiogenesis process. This observation is in drastic contrast to the traditional angiogenesis process contributed by surrounding endothelial progenitors that are triggered by cytokines and pro-angiogenic factors secreted from tumour-associated macrophages/neutrophils and tumour-associated fibroblasts [2] , [3] . Induction of tumour-derived endothelial differentiation by Twist1 is different from the vasculogenic mimicry mechanism [33] , [34] , which does not activate endothelial markers and may represent an incomplete differentiation towards the endothelial lineage. This induction of endothelial differentiation may be critical for tumour progression and metastasis since knockdown of either Jagged1 or KLF4 significantly decreases the in vitro or in vivo metastatic activity induced by Twist1 ( Fig. 8 ; Supplementary Figs 11c,d and 25c ). Inhibition of the angiogenesis process should be equally important to treat metastasis. Our results provide a mechanistic explanation why the Twist1-Jagged1-KLF4 axis reprograms HNC cells into endothelial cells and why it promotes angiogenesis that facilitates tumour progression and metastasis. This result is consistent with the reports that pluripotency factors regulate endoderm specification [19] and defects in the cranial vasculature are observed in Twist1-null mice [35] . Since knockdown of Twist1 in H1299 cells reverses the vascular marker expression pattern and decreases the haemoglobin levels in xenotransplanted mice ( Supplementary Figs 5c and 6 ), the same signalling pathway to mediate endothelial differentiation and vasculogenesis may be used in other tumour types. In contrast to its role in the generation of inducible pluripotent stem cells [16] , a distinct and detailed role of KLF4 in endothelial differentiation and vasculogenesis was demonstrated in this report. The regulation of KLF4 by Jagged1 shows the direct connection between the Notch pathway and KLF4. It should be pointed out that the regulation of tumour-initiating ability by KLF4 is independent of the pathways mediated by BMI1, which regulates the expression of CD44 surface marker and tumour sphere-formation ability as shown previously [24] . The downstream targets of KLF4 (for example, Wnt5A , CCND2 ) may control the stem-like property that contributes to the tumour-initiating ability. Finally, KLF4 contributes to Twist1-induced metastatic activity through an EMT-independent mechanism, suggesting that regulation of different targets (for example, motility genes) other than the typical EMT marker genes also contribute to the metastatic activity induced by Twist1 (ref. 29 ). All these results demonstrate the versatile role of KLF4 in Twist1-induced endothelial differentiation, stem-like property and metastasis. The knowledge gained from this report has therapeutic implications for combining γ-secretase inhibitors [32] with other chemotherapeutic agents to achieve additive tumour-killing effects in Twist1-overexpressing tumours, especially in head and neck tumours with a percentage (35–45%) expressing Twist1 [11] , [24] . Jagged1 has been shown to be a downstream target of Twist1, although the regulatory mechanism has not been demonstrated [36] . This report provides the mechanism of a direct regulation of Jagged1 expression by Twist1. Negative regulation of KLF4 by Notch signalling has been observed in intestinal epithelium or colorectal cancer cells [37] , [38] and these results are in favour of the tumour suppressor role of KLF4 in colorectal cancer cells [39] . In contrast to the tumour suppressor role of KLF4 in colorectal cancer cells/intestinal epithelium and pancreatic cancer [37] , [38] , [39] , [40] , [41] , other groups have demonstrated the oncogenic role of KLF4 in breast cancer and HNC [42] , [43] , [44] . These findings are consistent with our discovery that KLF4 plays an oncogenic role, especially in HNSCC [44] . In accordance with the general perception, KLF4 should be deemed as a context-specific oncogene or tumour suppressor gene, depending on the tumour cell types. Overall, our results propose that the Twist1-Jagged1-KLF4 axis induces tumour-derived endothelial differentiation inside tumours to produce a favourable tumour microenvironment in addition to the existing quiescent endothelial cells. A model to summarize this report is presented ( Fig. 9d ), in which tumour mesenchymal cells induced by Twist1 can migrate into tumour vasculature reprogrammed by the Jagged1-KLF4 axis to initiate the metastatic process. Cell culture The cell lines used include the human tongue squamous cell carcinoma cell lines OECM1 and SAS, human hypopharyngeal squamous cell carcinoma cell line FADU, lung cancer cell line H1299 and human embryonic kidney 293T cell line (all of them were obtained from American Type Culture Collection). The OECM1, SAS and FADU cell lines were used due to their low endogenous Twist1 levels and low metastatic activity (epithelial in nature). The H1299 cell line was used due to its higher Twist1 levels (mesenchymal in nature). The culture of primary head and neck tumour cells was performed by dissociating the tumour tissue in trypsin and collagenase, followed by culturing in RPMI medium containing 10% fetal bovine serum [24] . Informed consent was obtained from all subjects and the procurement of primary HNSCC tumours was approved by the Institutional Review Board (IRB) of Taipei Mackay Memorial Hospital. Protein extraction and western blot analysis For extraction of proteins from cell lines, cell lysis buffer (50 mM Tris, pH 7.5, 30 mM MgSO 4 , 8 mM EDTA, 2 mM dithiothreitol, 2% Triton X-100 and 0.2% SDS) containing protease inhibitors was used. Cell lysates were clarified by centrifugation at 13,000 r.p.m., 4 °C for 10 min. The protein content was determined by Bradford method (Bio-Rad Laboratories, Hercules, CA). For western blot analysis, 50–100 μg protein extracts from each clone were loaded to 10% SDS–PAGE gels and transferred to nitrocellulose filters. The filters were probed with different antibodies, and an anti-β-actin antibody was selected as a loading control. Signals were developed using an ECL chemiluminescence kit (Millipore, Billerica, MA). RNA extraction and quantitative real-time PCR Total RNA was isolated using Trizol reagent (Life Technologies, Carlsbad, CA) according to manufacturer’s recommendations. Single-stranded complementary DNA was synthesized by the RevertAid First Strand cDNA Synthesis Kit (Fermentas International, Burlington, Canada). Real-time PCR was performed on a Bio-Rad iCycler iQ PCR detection system according to the manufacturer’s instructions. The 2−ΔΔ C t method of relative quantification was used to estimate the copy number of gene expression [45] , and 18S was selected as an internal control. The sequences of the oligonucleotides for real-time PCR are shown in Supplementary Table 4 . Images of full blots can be seen in Supplementary Fig. 29 . In vitro migration/invasion and in vivo metastatic assays For in vitro migration/invasion assay, 8 μm pore size Boyden chamber was used. Cells (4 × 10 4 ) in 0.5% serum-containing RPMI were plated in the upper chamber and 15% fetal bovine serum was added to RPMI 1640 in the lower chamber as a chemoattractant. For invasion assay, the upper side of the filter was covered with Matrigel (BD Biosciences, San Jose, CA; 1:2 dilution with RPMI). After 12 h for migration assay or 24 h for invasion assay, cells on the upper side of the filter were removed, and cells that remained adherent to the underside of membrane were fixed in 4% formaldehyde and stained with Hoechst 33342 dye. The number of migrated cells was counted using a fluorescence microscope. Ten contiguous fields of each sample were examined using a × 40 objective to obtain a representative number of cells that migrated/invaded across the membrane. For in vivo tail vein metastasis assay, five 6-week-old female non-diabetic-severe combined immunodeficiency (NOD-SCID) mice received injection of 4 × 10 6 cells of different cell lines in 0.1 ml of phosphate-buffered saline (PBS) via the tail vein (six mice for each group). Four to 6 weeks after injection, mice were examined grossly at necropsy for the presence of metastases in internal organs such as lung tissue and lymph node area. Microscopic examination of metastases was performed on the cross-sections of formalin-fixed, paraffin-embedded lung tissues stained with H&E. The counting of metastatic lesions in the internal organ of each mouse was evaluated by gross and microscopic examination. Plasmids and stable transfection The Twist1 expression vector (Flag-CMV-Twist1 or pcDNA3-Twist1) was generated by inserting a 694-base pair fragment of the full-length Twist1 cDNA into the pFlag-CMV vector [11] or the pcDNA3 vector. The pcDNA3-Jagged1 was generated by inserting a 3,657-bp fragment of the full-length human Jagged1 cDNA into the HindIII/EcoRI sites of the pcDNA3 vector. The KLF4 expression vector was obtained from Dr S.C. Teng (National Taiwan University, Taiwan). Calcium phosphate transfection method by mixing calcium chloride and phophostate solution to generate plasmid precipitates was used for plasmid transfection [11] , [24] . Stable clones were generated by transfection of expression vectors or infection with lentivirus short hairpin RNA (shRNA) plasmids and selected by appropriate antibiotics. Transient transfection and luciferase assays The Jagged1 and KLF4 promoter regions were cloned and the reporter constructs are shown in Supplementary Tables 5 and 6 . Both the Jagged1 promoter mutant reporter construct and the KLF4 promoter mutant report construct were generated using site-directed mutagenesis. The reporter constructs were co-transfected into 293T cells using calcium phosphate transfection method with different expression vectors and an internal control plasmid. Luciferase assays were performed using the same amount of cell extracts and corrected for transfection efficiency using an internal control (β-gal or GFP) [11] , [24] . Standard and qChIP Cells were cross-linked [46] with 2% formaldehyde for 10 min and stopped by adding glycine to a final concentration of 0.125 M. Fixed cells were washed twice with Tris-buffered saline (TBS) (20 mM Tris, pH 7.5, 150 mM NaCl) and collected in 5 ml of SDS buffer (50 mM Tris, pH 8.0, 0.5% SDS, 100 mM NaCl, 5 mM EDTA and protease inhibitors). Cells were pelleted by centrifugation and suspended in 2 ml of immunoprecipitation (IP) buffer (100 mM Tris, pH 8.6, 0.3% SDS, 1.7% Triton X-100 and 5 mM EDTA). Cells were sonicated with a 0.25-inch diameter probe for 15 s twice using an MSE-soniprep 1,500 sonicator (setting 18). For each immunoprecipitation, 1 ml of lysate was precleared by adding 50 ml of blocked protein A beads (50% protein A-Sepharose, Amersham Biosciences; 0.5 mg ml −1 bovine serum albumin, 0.2 mg ml −1 salmon sperm DNA) at 4 °C for 1 h. Samples were spun, and the supernatants were incubated at 4 °C overnight with no antibody, immunoglobulin (Ig)G, anti-twist, anti-NOTCH-ICD, anti-KLF4 or anti-BMI1 antibody. Immune complexes were recovered by adding 50 ml of blocked protein A beads and incubated overnight at 4 °C. Beads were successively washed with (1) mixed micelle buffer (20 mM Tris, pH 8.1, 150 mM NaCl, 5 mM EDTA, 5% w/v sucrose, 1% Triton X-100 and 0.2% SDS), (2) buffer 500 (50 mM Hepes, pH 7.5, 0.1% w/v deoxycholic acid, 1% Triton X-100, 500 mM NaCl and 1 mM EDTA), (3) LiCl detergent wash buffer (10 mM Tris, pH 8.0, 0.5% deoxycholic acid, 0.5% Nonidet P-40, 250 mM LiCl and 1 mM EDTA) and (4) TE buffer (10 mM Tris and 1 mM EDTA) and then eluted with 1% SDS and 0.1 M NaHCO 3 . NaCl (5 M; 20 ml) was added to the elutes, and the mixture was incubated at 65 °C for 5 h to reverse the cross-linking. After digestion with proteinase K, the solution was phenol/chloroform extracted and ethanol precipitated. For standard ChIP, DNA fragments were resuspended in 50 μl of water and 5 μl was used in a PCR reaction for 30 cycles. For qChIP analysis, DNA fragments were resuspended in 400 μl of water and 5 μl was used by real-time PCR. Each sample was calculated as the percentage of input sample. The sequences of PCR regions and primers used in ChIP assay are listed ( Supplementary Tables 5–7 ). The source and concentration of the antibodies used are listed ( Supplementary Table 8 ). Immunofluorescence staining and flow cytometry For immunofluorescence staining, cells on glass coverslips or chamber slides were fixed with 4% paraformaldehyde and permeabilized with 0.5% Triton X-100. After washing three times for 10 min with PBS, fixed cells or slides were blocked with blocking buffer (PBS, 0.1% Tween-20, with 3% goat serum) for 1 h and incubated with primary antibody diluted in blocking buffer overnight at 4 °C. After washing three times with PBS for 10 min, the fixed cells were treated with the appropriate secondary antibody (fluorescein isothiocyanate-conjugated anti-mouse IgG or rhodamine-conjugated anti-rabbit IgG; Sigma) that was diluted in a blocking buffer for 1 h at room temperature. Finally, the fixed cells were washed three times for 10 min with TBS, and their nuclei were counterstained, mounted and observed by fluorescence microscope or confocal microscope. The paraffin-embedded tissue specimens from patient samples and mouse samples were de-paraffinized in xylene, rehydrated through graded ethanol and rinsed in PBS buffer. Antigen retrieval processes were then performed by pressure cooker at 1.2 atm for 15 min with 1 mM sodium citrate buffer (pH 6.0) and then incubated with 20 μg ml −1 Proteinase K in TE buffer at 37 °C for 20 min. These slides would be used for immunofluorescence staining by using hCD31, CD144, Twist1 and GFP antibodies, the detailed antibody information is shown in the Supplementary Table 8 . The characterizations of the specificity of endothelial marker antibodies such as CD31 and CD144 are shown ( Supplementary Fig. 28b ). The CD31 antibody is human specific since staining of mouse tissue was negative. The CD144 antibody could stain both human and mouse CD144. Informed consent was obtained from all subjects and the usage of patient samples was approved by the IRB of Taipei Mackay Memorial Hospital. To analyse the expression of specific cell surface markers, cells were resuspended and incubated with fluorescein isothiocyanate-conjugated anti-CD44 antibody, PE-conjugated anti-CD31 antibody and PE-conjugated anti-CD144 antibody, respectively. The stained cells were evaluated using a FACSCalibur flow cytometer (BD Biosciences). At least 10,000 cells were analysed per sample and each staining experiment was repeated four times. CELLQuest analysis software was used for fluorescence determination and data analysis. Flowjo was used to generate the dot plots. Lentiviral infection Lentivirus containing shRNAs expressed in a lentiviral vector (pLKO.1-puro) was generated in 293T cells as previously described [47] . Plasmids pLKO-Luciferase-i, pLKO-KLF4-i-3, pLKO-KLF4-i-934, pLKO-GFP and packaging plasmid pCMVΔR8.91 were obtained from S.C. Teng (National Taiwan University, Taiwan). Plasmids pLKO-BMI1-i-2 and pLKO-BMI1-i-3 were provided by National RNAi Core Facility of Academia Sinica, Taipei, Taiwan. For lentivirus production, 293T cells were transfected with 15 μg pLKO.1-puro lentiviral vectors expressing different shRNAs along with 1.5 μg of envelope plasmid pMD.G and 15 μg of packaging plasmid pCMVΔR8.91. Virus was collected 48 h after transfection. To prepare KLF4- or Bmi1-knockdown cells, OECM1-Twist1 cells were infected with lentivirus for 24 h, and stable clones were generated by selection with appropriate antibiotics. The sequences for the lentivirus are shown in Supplementary Table 4 . 2.5-Dimensional tube-formation assay For experiments in which [48] cells were cultured on top of the Matrigel, 50 μl growth factor reduced Matrigel was plated in eight-well chamber slides. The chambers were then incubated at 37 °C for 30 min to allow Matrigel to polymerize. Cells (1 × 10 4 ) were added onto the top of the Matrigel in each well. After incubation for 5 days, the slides were examined for endothelial tubes using light microscope. Five random images per well were quantified by the MetaMorph Imaging System, a digital imaging software to analyse biological images. The angiogenesis tube formation module was used to analyse tube-formation activity. The image was run through the software to identify tubes or nodes. A pixel is a single point in a graphic image as a unit of measurement. 3D tube-formation assay For 3D culture, tumour cells were resuspended in 5 mg ml −1 growth factor reduced Matrigel (BD Biosciences) on ice. Cells (1 × 10 4 ) per each well were seeded in eight-well chamber slides and allowed to polymerize at 37 °C for 30 min followed by adding 10% serum-containing MCDB131 culture medium onto the top of the wells. The chambers were then incubated at 37 °C. After incubation for 5 days, the slides were used for DiI-AcLDL uptake analysis and immunofluorescence assay. DiI-AcLDL uptake analysis The functional assay for endothelial cells was performed by incubation of cells with 10 μg ml −1 of DiI-AcLDL (Molecular Probes, Invitrogen) for 4 h followed by observation by fluorescence microscope. A picture with 3D tumour formation assay was usually accompanied with the LDL uptake picture to indicate the presence of cell clones tested. Subcutaneous implantation and haemoglobin quantification For in vivo monitoring of tumour-associated angiogenesis, 1 × 10 6 cells of different cell lines in 0.1 ml Matrigel were injected under the abdominal skin of 6-week-old female Balb/c nude mice. After tumour formation (4–6 weeks after injection), animals were killed and matrigel implants were collected, weighed and fixed in 4% paraformaldehyde for IHC analysis or in PBS for haemoglobin quantification. Haemoglobin contents of matrigel implants were measured using a Drabkin’s reagent kit (Sigma) [48] . The tissue was transferred into the Eppendorf containing 0.5 ml PBS buffer under overnight incubation at 37 °C to lyse red blood cells and release haemoglobin. The tissue samples were homogenized and spun down to collect the clear supernatant. Samples (50 μl) of tissue supernatant were added to 1 ml Drabkin’s reagent and then incubated for 15 min at room temperature. Absorbance of each sample was measured at 540 nm. The results are divided by tissue weight and expressed as haemoglobin concentration (mg mg −1 ). Drug treatment of xenografted mice In the xenotransplanted tumour model, the OECM1-Twist1 cells (2 × 10 6 ) in 0.2 ml PBS were injected into the right lateral flank of 6-week-old female Balb/c Nude mice. Treatment was started when the tumours grew to certain size. Mice were treated once a week by intraperitoneal injections of 10 mg kg −1 cetuximab (Merck KGaA, Darmstadt, Germany) or 100 mg kg −1 DAPT [30] (Selleck Chemicals., Houston, USA) or both together. The tumour size of each group was monitored and measured every week. Tumour volume (mm 3 ) was estimated according to the formula length × (width) 2 × 0.5 in mm 3 . Tumour sphere formation Cells (1 × 10 3 ) were seeded [24] and incubated with serum-free medium composed of DMEM/F-12 (Thermo Fisher Scientific, USA), N2 supplement (Thermo Fisher Scientific), 10 ng ml −1 human recombinant basic fibroblast growth factor (bFGF) (R&D Systems, USA) and 10 ng ml −1 epidermal growth factor (EGF) (R&D Systems, USA) in a 24-well plate. The spheroids were resuspended to form secondary and tertiary spheroids. Only the tumour spheres with a size >100 μm were counted. The number of spheroids was counted after 14 days. Tissue microarray construction A high-density tissue [49] microarray was constructed using formalin-fixed, paraffin-embedded specimens of HNSCC patient samples’ H&E-stained sections that were made from each paraffin block to define representative tumour regions. Tissue cylinders with a diameter of 0.6 mm were punctured from these regions in the paraffin block and arrayed into a recipient block using the tissue chip microarrayer (Beecher Instruments, Silver Spring, MD). The recipient block was serially cut into 5-μm sections on silanized slides (Dako, Glostrup, Denmark). Informed consent was obtained from all subjects and the protocol was approved by the IRB of Taipei Veterans General Hospital. In situ hybridization The paraffin-embedded tissue specimens were de-paraffinized in xylene, rehydrated through 100, 90, 70, 50% ethanol and rinsed in PBS buffer. Antigen retrieval processes were then performed twice by pressure cooker at 1.2 atm for 15 min with target retrieval solution (#S1700, Dako, Denmark) and then blocked with 0.3% hydrogen peroxide for 30 min. Biotinylated probes (20 μl) for general screening (HPV 6, 11, 16, 18, 30, 31, 33, 45, 51, 52; #Y1404, DAKO) were applied on separate specimen and were covered with coverslips. Denaturation of DNA was performed at 92 °C for 5 min in an oven. Hybridization was performed in a humid chamber at 37 °C overnight. After washing, the GenPoint Kit (#K0620; DAKO) was used according to the manufacturer’s instruction. IHC, scoring and validation of antibodies The sample processing and [11] , [24] , [46] IHC procedure for determining the immunoreactivity of Twist1, Jagged1 and KLF4 were described as the following. The paraffin-embedded tissue specimens were de-paraffinized in xylene, rehydrated through 100, 90, 70, 50% ethanol and rinsed in PBS buffer. Antigen retrieval processes were then performed by pressure cooker at 1.2 atm for 15 min with 1 mM sodium citrate buffer (pH 6.0) and then blocked with 3% hydrogen peroxide for 30 min. The specimens were incubated with primary antibodies in 5% BSA buffer in a humidity chamber overnight at 4 °C. Detection of the staining was used by the Super Sensitive Non-Biotin Polymer HRP Detection System according to the manufacturer’s instructions (BioGenex, San Ramon, CA). The immunoreactivity of Twist1, Jagged1 and KLF4 was graded from 0 to 3+ (0, no staining; 1+, 1–25%; 2+, 26–50%; 3+, >50% nuclear staining) according to nuclear expression, and only 3+ (>50% nuclear staining) was considered as a positive IHC result. All IHC staining was independently scored by two experienced pathologists. If there was discordance with IHC scoring, a pathologic peer review will be performed to consolidate the result into a final score. The pathologists scoring the IHC were blinded to the clinical data. The interpretation was performed in five high-power views for each slide, and 100 cells for each view were counted for analysis. Validation of Twist1 antibody was described [11] . Validation of antibodies against Jagged1 and KLF4 was performed from various overexpression and knockdown experiments (for example, Jagged1 from Supplementary Figs 11a,b and 12b,c ; KLF4 from Fig. 6a ; Supplementary Fig. 21b ) as well as from the manufacturer’s protocols. Higher-magnification photos of certain images can be seen in Supplementary Fig. 30 . Statistical analysis The independent Student’s t -test was used to compare the continuous variables between two groups, and the χ 2 test was applied for comparison of dichotomous variables in tables. The control groups of all the statistical analyses were specified in the figure legends. The level of statistical significance was set at 0.05 for all tests unless specified. Accession codes: The raw data of microarray (H1299 control versus H1299-Twist1-si) were deposited to GenBank in MIAME format and the accession number is GSE57756 . How to cite this article: Chen, H.-F. et al. Twist1 induces endothelial differentiation of tumour cells through the Jagged1-KLF4 axis. Nat. Commun. 5:4697 doi: 10.1038/ncomms5697 (2014).